Strong Schottky barrier reduction at Au-catalyst/GaAs-nanowire interfaces by electric dipole formation and Fermi-level unpinning Nanoscale contacts between metals and semiconductors are critical for further downscaling of electronic and optoelectronic devices. However, realizing nanocontacts poses significant challenges since conventional approaches to achieve ohmic contacts through Schottky barrier suppression are often inadequate. Here we report the realization and characterization of low n -type Schottky barriers (~0.35 eV) formed at epitaxial contacts between Au-In alloy catalytic particles and GaAs-nanowires. In comparison to previous studies, our detailed characterization, employing selective electrical contacts defined by high-precision electron beam lithography, reveals the barrier to occur directly and solely at the abrupt interface between the catalyst and nanowire. We attribute this lowest-to-date-reported Schottky barrier to a reduced density of pinning states (~10 17 m −2 ) and the formation of an electric dipole layer at the epitaxial contacts. The insight into the physical mechanisms behind the observed low-energy Schottky barrier may guide future efforts to engineer abrupt nanoscale electrical contacts with tailored electrical properties. Electrical contacts between metals and semiconductors are fundamentally important for semiconductor devices [1] , [2] , [3] . Shrinking their dimensions poses significant challenges because the properties of metal/semiconductor contacts at the nanoscale may differ significantly from those of their macroscopic counterparts, and the same approaches to control these properties are not always suitable at the nanoscale [4] , [5] , [6] , [7] , [8] , [9] . In particular, standard approaches to realize ohmic contacts by suppressing Schottky barriers through heavy doping and/or varying semiconductor chemical composition in the contact region by, for example, an alloy formation [10] are inadequate at the nanoscale. One promising type of nanoscale electrical contact that may help alleviate this problem is the epitaxially formed contact between a semiconductor nanowire (NW) and the corresponding metal-catalyst nanoparticle used to grow it. Such contacts have been reported to exhibit a reduced Schottky barrier influence on the contact properties [11] , [12] , [13] . Possible mechanisms behind this interesting behaviour were attributed to an increased role of contact periphery effects compared with microscale contacts [11] , midgap states induced at the contact interface [12] and Fermi-level unpinning at the contact interface [13] . However, the origin of the observed reduction of the Schottky barrier influence is still far from fully understood. For the specific case of nanocontacts formed at Au-catalyst/GaAs-NW interfaces—such systems are particularly interesting because of their technological importance [14] —a reduction of the n -type Schottky barrier height from the normally observed value of 0.9 to 0.52 eV was reported [13] . In that case, the Schottky barrier lowering was attributed to an alleviated Fermi-level pinning. However, because of limited precision in contacting the Au-catalyst in the experiment there was also an overlap between the thin film electrode and the NW segment below the Au catalyst, which makes the interpretation of the results more challenging as this overlap may, for example, change the field distribution in the semiconductor region. Furthermore, it was unclear whether the nanocontact properties could be further improved beyond what was previously reported [13] , [14] . It therefore remains unclear whether and how low-energy Schottky barriers can be realized at metal-catalyst/NW interfaces. Here we demonstrate and characterize by high-precision selective contacts defined by electron beam lithography (EBL) a surprisingly low, ~0.35 eV, n -type Schottky barrier that is formed directly and solely at the abrupt epitaxial interface between an Au-In alloy catalytic tip (Au catalyst later in the text) and a GaAs NW. The strong reduction of the Schottky barrier height (considerably lower barrier than the typically observed 0.9 eV for ordinary Au/GaAs Schottky contacts and the lowest barrier observed at Au/GaAs interfaces to date) occurs because of a combination of reduced density of pinning states and the formation of an electric dipole layer at the Au-catalyst/GaAs-NW interface owing to the termination of the GaAs NW by As atoms. Insight about these barrier-lowering mechanisms may enable Schottky barrier height control and low-ohmic abrupt electrical contacts to be formed at metal–semiconductor–nanostructure interfaces without the need for annealing or contact doping, otherwise limiting factors in rapid downscaling of nanodevices. Experimental design To obtain a comprehensive understanding of the mechanisms behind the Schottky barrier formation at metal-catalyst/NW interfaces, we considered two different types of NWs, as well as two independent characterization methods. The A series comprised Au-catalyst/GaAs/InGaAs/InAs-NW heterostructures with 90 nm diameter, grown by chemical beam epitaxy (CBE) on InAs (111)B substrates. The Au catalysts were alloyed with In during the NW growth. These NWs were probed with EBL-defined contacts and characterized by current–voltage ( I–V ) measurements at different temperatures and under illumination. More details on the NW growth can be found in Methods and elsewhere [15] . The B series comprised Au-catalyst/GaAs-NWs with 95 nm diameter, grown by metal organic vapour phase epitaxy (MOVPE) on GaAs (111)B n -type substrates. The Au catalysts were alloyed with In before the NW growth. These NWs were used for complementary I–V measurements at room temperature by direct contacting of the Au-catalyst particles with the tip of a scanning tunnelling microscope (STM) to verify the observed Schottky barrier height. More details on the NW growth can be found in Methods and elsewhere [16] . Both types of NWs (series A and B ) grew perpendicular from the substrate indicating that the epitaxial contact was formed at the Au-catalyst/GaAs (111)B NW interface. The chosen NW design in our study was motivated by the following: first, the selective electrical contacting to the Au-catalyst was realized with a high-precision EBL alignment scheme, which ensured that electron transport occurred solely through the epitaxial Au-catalyst/GaAs-NW interface. The EBL-defined contacts also enabled detailed characterization, including I–V measurements at different temperatures and under light excitation. Second, the heterostructure NW design implemented for the NWs in series A allowed the formation of electrical contacts to the Au-catalyst/GaAs-NW interface from the NW side through an ohmic contact to the InAs NW segment [17] via a graded InAs/InGaAs/GaAs heterojunction. In this way, deleterious effects from parasitic electrical contacts were eliminated. Third, the NW diameter used in our experiments allows a direct comparison with previous studies [11] , [13] , while at the same time ensuring that quantum mechanical confinement effects do not significantly influence the observed phenomena. Fourth, the experimental design ensured that a wide enough potential barrier was formed at the Au-catalyst/GaAs-NW interface to avoid any tunneling effects. Finally, the alloying of the Au catalyst with In in our experiments was done because In/GaAs-alloyed contacts are known to exhibit a low Schottky barrier height of merely 0.03 eV (ref. 18 ). Series A NW characterization To elucidate the structural and elemental composition of the heterostructure NWs from series A , we performed a transmission electron microscopy (TEM) and X-ray energy-dispersive spectroscopy (XEDS) analysis ( Fig. 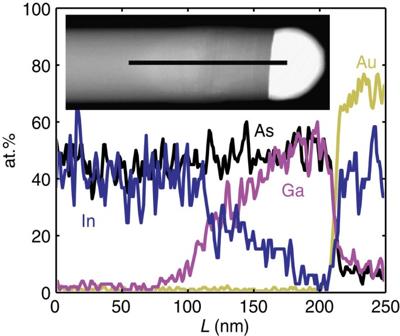Figure 1: XEDS line scan for a seriesAheterostructure NW. The XEDS scan was done along the line indicated in the TEM micrograph (inset). Note that the line scan shows an approximate element distribution in the NW as the XEDS count normalization needs to be done differently in different regions. XEDS point measurements revealed a 31±1 at.% In content in the catalytic particle, whereas the Ga and As contents were found to be below the detection limit (1–2 at.%;Supplementary Table 1). 1 ); more details on the NW inspection with TEM can be found in Methods and Supplementary Table 1 . The TEM image reveals that an abrupt contact is formed between the NW and the metal particle (inset of Fig. 1 and Supplementary Fig. 1 ). The XEDS analysis shows that the length of the pure GaAs segment right under the Au catalytic particle was ~25 nm, while the graded InGaAs segment was ~75 nm with a smooth transition from pure GaAs to pure InAs. Note that the line scan presented in Fig. 1 shows an approximate element distribution in the NW as the XEDS count normalization needs to be done differently in different regions. Figure 1: XEDS line scan for a series A heterostructure NW. The XEDS scan was done along the line indicated in the TEM micrograph (inset). Note that the line scan shows an approximate element distribution in the NW as the XEDS count normalization needs to be done differently in different regions. XEDS point measurements revealed a 31±1 at.% In content in the catalytic particle, whereas the Ga and As contents were found to be below the detection limit (1–2 at.%; Supplementary Table 1 ). Full size image The XEDS point measurements revealed a 31±1 at.% In content in the catalytic particle, whereas the Ga and As contents were found to be below the detection limit of 1–2 at.% ( Supplementary Table 1 ). No GaAs shell was observed around the InAs segment. These results demonstrate that the Au catalysts in our series A NWs were alloyed with In only. Furthermore, there was no Au-alloying of the GaAs and thus, an abrupt contact was formed between the NW and the metal particle. To enable detailed electrical characterization of the catalyst/NW interfaces, we formed electric contacts selectively to the catalytic particle using EBL (inset of Fig. 2 ). To the best of our knowledge, this is the first time a NW catalyst particle has been selectively contacted by EBL. It was made possible owing to a high-precision alignment before the EBL exposure, which allowed a control of the electric contact position with 10–20 nm precision (more details on electrical contact formation can be found in Methods and elsewhere [17] ). 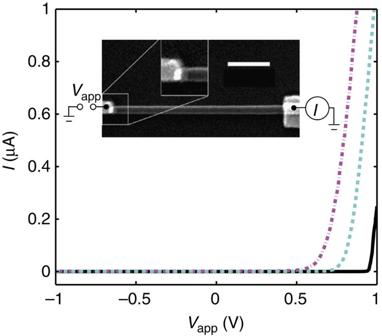Figure 2:I–Vcharacteristics for a heterostructure NW device from seriesA. I-Vcharacteristics recorded at 4.2 K (black solid line), 300 K (turquoise dashed line) and 410 K (magenta dash-dotted line). The inset shows a scanning electron microscope (SEM) image of the measured device and the schematic electrical circuit set-up for the measurements. Scale bar, 500 nm. Zoomed region shows the selective electrical contact formed to the catalytic particle. Figure 2: I–V characteristics for a heterostructure NW device from series A . I-V characteristics recorded at 4.2 K (black solid line), 300 K (turquoise dashed line) and 410 K (magenta dash-dotted line). The inset shows a scanning electron microscope (SEM) image of the measured device and the schematic electrical circuit set-up for the measurements. Scale bar, 500 nm. Zoomed region shows the selective electrical contact formed to the catalytic particle. Full size image Electrical measurements on the series A NWs revealed highly asymmetric, rectifying I–V characteristics at different temperatures indicating electron transport governed by a thermionic emission (TE) over an n -type potential barrier ( Fig. 2 , inset shows a schematic picture of the electrical circuit used in the measurements). The two possible positions along the NW at which a potential barrier may be formed are at the Au-catalyst/GaAs-NW interface and in the GaAs/InGaAs-NW segment. As we will show in the following analysis, the relevant potential barrier determining the electron transport at large reverse bias is formed at the Au-catalyst/GaAs-NW interface. A model based on TE of electrons is used to evaluate the properties of this potential barrier. According to TE theory, the I–V characteristics for V app <− 3 kT/q are described by: where V app is the applied voltage, I is the current through the device, A is the effective contact area between the catalytic particle and the NW, A * is the Richardson constant and q ϕ E ( V app ) is the effective voltage-dependent energy barrier height (for details see Methods and elsewhere [1] , [19] ). Arrhenius plots ( Fig. 3b ) were extracted from temperature-dependent I–V measurements ( Fig. 3a ) and analysed using equation (1). 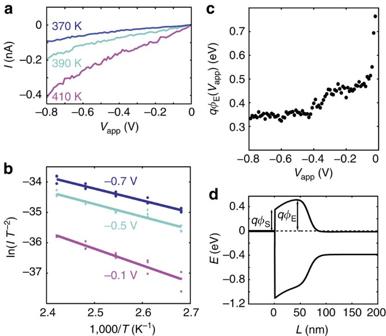Figure 3: The Schottky barrier height extraction for a heterostructure NW device from seriesA. (a)I-Vcharacteristics at different temperatures in the reverse bias region. (b) Arrhenius plots extracted fromI–Vcurves measured in the temperature range 370–410 K. (c) The extracted effective voltage-dependent energy barrier heightqϕE(Vapp) plotted versus applied biasVapp. Negative bias corresponds to a reverse-biased Schottky contact;cf.the inset inFig. 2. This analysis is only valid forVapp<−3kT/q, which explains the large scattering observed close to zero bias. (d) Band diagram reconstruction of the studied NW heterostructure at thermal equilibrium. HereqϕEindicates the energy barrier height at zero bias. Figure 3c shows the extracted barrier height qϕ E ( V app ) for different bias V app . The results reveal that the barrier height for small applied bias ( V app >−0.1 V, negative bias applied to the Au particle with respect to the grounded InAs segment of the wire) is ~0.5 eV, while for large bias ( V app <−0.4 V) the barrier height saturates at 0.35±0.03 eV. Since equation (1) is valid only for V app <− 3 kT/q (~0.08 V), the extracted values close to zero bias are not accurately described by equation (1) and therefore the scattered points in this region are not meaningful. Figure 3: The Schottky barrier height extraction for a heterostructure NW device from series A . ( a ) I-V characteristics at different temperatures in the reverse bias region. ( b ) Arrhenius plots extracted from I–V curves measured in the temperature range 370–410 K. ( c ) The extracted effective voltage-dependent energy barrier height q ϕ E (V app ) plotted versus applied bias V app . Negative bias corresponds to a reverse-biased Schottky contact; cf. the inset in Fig. 2 . This analysis is only valid for V app <− 3 kT/q , which explains the large scattering observed close to zero bias. ( d ) Band diagram reconstruction of the studied NW heterostructure at thermal equilibrium. Here q ϕ E indicates the energy barrier height at zero bias. Full size image To interpret these results we reconstructed the band diagram shown in Fig. 3d . As input for this reconstruction, we used parameters known for this type of NWs and the barrier heights extracted from our experiments at V app >−0.1 V and V app <−0.4 V (for details see Methods and elsewhere [20] ). The results show that the entire GaAs/InGaAs segment is depleted from free carriers. As seen in the diagram, the potential barrier that forms at thermal equilibrium exceeds the n -type Schottky barrier height, q ϕ S . The reason for this is that q ϕ S <q ϕ GaAs –q χ GaAs , where q ϕ GaAs is the work function and q χ GaAs is the electron affinity of the GaAs NW segment. Therefore, a negative V app has to be applied to reach conditions where q ϕ S limits electron transport. We interpret the flat region for V app <−0.4 V ( Fig. 3c ) as the region where the electron transport is determined by the Schottky barrier between the Au catalyst and GaAs NW for which we extract q ϕ S =0.35±0.03 eV. This value is considerably smaller than 0.9 eV known for abrupt n -type bulk Au/GaAs Schottky contacts [21] , [22] . In fact, to the best of our knowledge, this is the smallest Schottky barrier height ever reported for Au/GaAs interfaces. An important comment to this analysis is that the effective contact area A between the Au catalyst and GaAs NW most likely depends on the applied bias [23] V app owing to self-gating effects [24] in combination with a surface depletion [23] , [25] due to NW surface oxidation [26] , [27] . However, such effects will not affect the extracted barrier height, as evident from equation (1) as well as from the saturation of the barrier height observed in Fig. 3c . The band diagram in Fig. 3d represents the potential profile along the core of the Au-catalyst/NW that determines the thermionic current [3] . This one-dimensional core profile is realistic also if one considers three-dimensional boundary conditions, for example, a Fermi-level position on the sidewall surface of the NW <0.7–0.9 eV below the conduction band (values known for oxidized GaAs surfaces) [28] . The soft reverse I–V characteristics observed ( Fig. 3a ) can also be understood from this model [25] as a self-gating effect [24] where the reverse current continues to increase with bias ( Fig. 3a ), although the effective potential barrier q ϕ E (V app ) saturates for V app <−0.4 V ( Fig. 3d ). The increasing reverse current results from an increase of the effective cross-section of the saddle point, which is decoupled from the Schottky barrier height in our analysis (for details see Methods). It is also important to note that our interpretation of the experimental results is based on the assumption that TE is the dominant electron transport mechanism. If another current component, comparable to the TE current in magnitude, existed then the extracted barrier height could be misestimated. Indeed, the following current components besides TE current can be observed in a metal–semiconductor junction [1] : (i) quantum mechanical tunnelling through the barrier and (ii) electron-hole generation-recombination. The NW design in our case was chosen in such a way that TE dominates. The InAs segment is unintentionally degenerately n -type doped (electron concentration ~10 17 cm −3 ) [29] , while the GaAs segment is non-degenerately p -type doped (with the same doping concentration) [30] . The length of the GaAs segment ensures a complete depletion of free carriers and that the potential barrier formed suppresses any tunnelling effects. Moreover, the GaAs segment creates an efficient potential barrier for both electrons and holes and the generation-recombination currents due to deep levels in Au/GaAs Schottky diodes are typically negligible [31] . Indeed, at 4.2 K we did not observe any current (<10 −12 A) for the voltage range used in our analysis, indicating that there is no tunnelling current or other currents at low temperature. However, temperature is known to have a profound effect on thermally activated tunnelling (thermionic field emission; TFE) and generation-recombination currents [32] . Linear characteristics in the Arrhenius plots in Fig. 3b indicate that TE dominates in our case since TFE and generation-recombination currents exhibit different temperature dependences [10] and any significant contribution to the TE current would result in nonlinear characteristics in the Arrhenius plots. Series B NW characterization To verify that the observed Schottky barrier height is not specific only to NWs from series A , and as a validation of the Schottky barrier height analysis, we carried out complementary I-V measurements at 300 K on NWs from the B series using STM under ultra-high vacuum conditions (see Methods and elsewhere [33] for details). 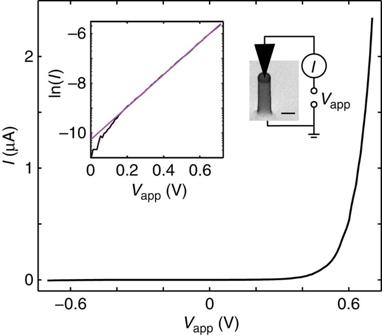Figure 4:I–Vcharacteristics for a seriesBNW. STM-based measurements ofI–Vcharacteristics for a nominally undoped GaAs NW at 300 K. The left inset shows a semi-log plot with a linear fit in the forward bias region (magenta line). The right inset shows an SEM micrograph of a typical NW together with the schematic electrical circuit used for the measurements. Scale bar, 100 nm. Figure 4 shows typical I–V data recorded with the STM on nominally undoped NWs with 95 nm diameter and ~500 nm length. The highly asymmetric, rectifying I–V curve ( Fig. 4 ) indicates that the electron transport is mainly determined by an n -type potential barrier. The red line in the inset shows a linear least-square fit of the semi-log I versus V app for V app >> kT/q . Extrapolating this line to V app =0 gives the saturation current I s , which was used to calculate q ϕ S according to: Figure 4: I–V characteristics for a series B NW. STM-based measurements of I–V characteristics for a nominally undoped GaAs NW at 300 K. The left inset shows a semi-log plot with a linear fit in the forward bias region (magenta line). The right inset shows an SEM micrograph of a typical NW together with the schematic electrical circuit used for the measurements. Scale bar, 100 nm. Full size image From this analysis we obtained q ϕ S =0.32±0.04 eV for NWs from series B , which is in good agreement with the q ϕ S deduced for the NWs in the A series discussed above (see Methods and elsewhere [1] , [19] for more details). It is also important to note that in this case we observe a large ideality factor n =2.6±0.2. Traditionally, the ideality factor was used to determine the deviation of electron transport from TE. However, as recognized already in the 1990s [3] , the ideality factor cannot be used for the determination of transport mechanisms, especially for NW geometries [25] . Our experimental design ensured that the effect of TE dominates over TFE since kT >> E 00 , where E 00 is a property of the semiconductor indicating how efficient tunnelling is in the semiconductor [3] . For the studied NWs, E 00 <7 meV (since the NW geometry increases the depletion region [11] , [26] ) while the measurements were done at room temperature ( kT =26 meV). Furthermore, a theoretical value of the expected low-bias differential conductance for TE [11] given by at 300 K with A *=7 A cm −2 K −2 and q ϕ S =0.35 eV yields 32 A V −1 cm −2 . This value is in good agreement with the experimental value of 30 A V −1 cm −2 deduced from our STM measurements. We therefore attribute the observed large ideality factor to surface depletion [23] , [25] due to NW surface oxidation [26] , [27] , an effect that we discussed above for NWs from series A . Mechanisms responsible for the low Schottky barrier To elucidate the physics behind this surprisingly low Schottky barrier, we will discuss several mechanisms that could be responsible for this result. First, the low barrier height observed in our experiments are not caused by annealing because the interface between the epitaxial Au-catalyst/GaAs-NW is abrupt according to TEM/XEDS, in contrast to the non-uniform Au diffusion into GaAs previously observed after annealing at 350 °C (ref. 14 ). This annealing resulted in a high dislocation density in the GaAs and the lowest-to-date barrier height for macroscopic Au/GaAs n -type Schottky contacts of ~0.5 eV. Second, a reduced Fermi-level pinning was previously suggested as a possible cause for lowering Schottky barriers at metal-catalyst/NW interfaces [13] . We suggest this effect to play a major role in our case since our observations do not fit the empirically known behaviour for abrupt metal contacts to n -type GaAs where the Schottky barrier depends on the metal work function q ϕ M according to q ϕ S =0.49+0.074 q ϕ M (refs 34 , 35 ). In case of pure Au ( q ϕ M =5.31 eV (ref. 36 )) in contact with GaAs, the corresponding Schottky barrier is expected to amount to q ϕ S(Au) =0.88 eV. Possible effects of In mixing in the Au catalyst also cannot explain the lowering since q ϕ In =4.12 eV (ref. 36 ), which corresponds to q ϕ S(In) =0.79 eV for a pure In contact to GaAs. A reduced density of interface pinning states was previously suggested to be responsible also for interface Fermi-level unpinning in GaAs grown at low temperature [37] . However, our observations cannot be explained solely by a reduced density of pinning states because a comparison with an ideal Schottky model reveals higher barrier values than we observe. According to the ideal Schottky model [1] , which does not consider Fermi-level pinning, the n -type Schottky barrier height depends on the contact metal work function as q ϕ S = q ϕ M –q χ, where q χ is the semiconductor affinity, q χ GaAs =4.07 eV (ref. 38 ). The work function of solid solution alloys can be described by a simple mixture rule of the surface composition: q ϕ AuIn = qx Au ϕ Au + qx In ϕ In , where x i is the atomic fraction of element i at the surface [39] . This expression yields q ϕ AuIn =4.96 eV for a 30 at.% In content in the Au catalyst, which corresponds to q ϕ S(AuIn) =0.89 eV, a considerably higher value than we observe in our experiments. We explain the barrier lowering by a reduced density of pinning states combined with a formation of an electric dipole layer. The dipole layer is formed because of the termination of the GaAs NW by As atoms at the contact interface with the Au-catalyst. The Au-catalyst/GaAs-NW interface studied in this work had a (111)B structure as the NWs grew vertically on (111)B substrates. This (111)B GaAs plane has only As atoms at the interface. Since As atoms in contact with an Au catalyst have higher electronegativity than Ga atoms, an interfacial electric dipole layer is formed with a dipole moment μ pointing towards the semiconductor NW and an associated electric field E directed towards the Au catalyst ( Fig. 5 ). This electric field leads to an effective reduction of the Schottky barrier. The ideal Schottky model ( Fig. 5a ) predicts the Schottky barrier for the In-alloyed Au-catalyst/GaAs-NW interface of q ϕ S(AuIn) =0.89 eV discussed in the previous paragraph. The electric field associated with the dipole layer leads to a step in the potential energy at the interface ( Fig. 5b ), which shifts the conduction band edge of the GaAs NW below the Fermi level in the Au-catalyst particle by an amount q Δ=0.33 eV (see Methods for details). If we now assume that pinning states at the interface account for the potential energy qd ϕ States =q ϕ S + q Δ=0.68 eV, we can estimate a density of surface states at the Au-catalyst/GaAs interface of ~10 17 m −2 (see Methods for details). Remarkably, as it was previously shown [40] , this density of surface states implies that the Fermi level is no longer pinned at the interface, and both the surface states and the work function difference will affect the Schottky barrier height. 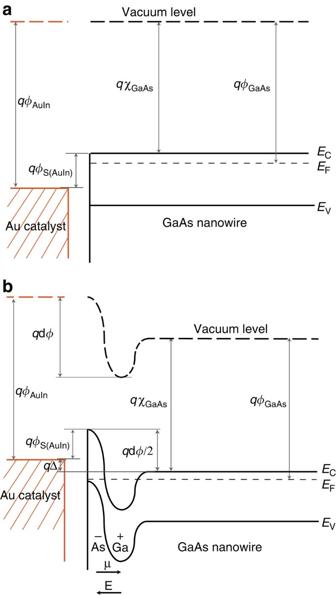Figure 5: Energy band alignment of an isolated Au catalyst andn-type GaAs (111)B NW. (a) Ideal Schottky model. (b) Ideal Schottky model with included electric surface dipole layer formed because of As termination of the GaAs NW. Figure 5: Energy band alignment of an isolated Au catalyst and n -type GaAs (111)B NW. ( a ) Ideal Schottky model. ( b ) Ideal Schottky model with included electric surface dipole layer formed because of As termination of the GaAs NW. Full size image Based on these arguments, we thus conclude that our observation of the drastic decrease in Schottky barrier height in our NW systems is caused by the combined effects of a reduced density of pinning states (~10 17 m −2 ) at the epitaxially formed Au-catalyst/GaAs-NW interface and an electric dipole layer formation at the same interface because of the termination of the GaAs NW by As atoms. It is known that GaAs NWs often have two crystal phases with different band gap alignment and sizes [41] , [42] . In our samples the presence of two crystal phases is manifested by stacking faults ( Supplementary Fig. 1 ) and it is not possible to conclude whether the Schottky contact in our case was formed with a Zinc blende or with a Wurtzite phase of GaAs. For bulk GaAs, the Zinc blende phase is the only phase possible and thus essentially all Schottky barrier height studies to date (except perhaps a recent report where the phase influence is not discussed [13] ) were done for this crystal phase. However, as recently shown by different groups [41] , [42] , the difference in band gap alignment and band gap size is below 0.1 eV, which is much smaller than the Schottky barrier reduction observed in our case and comparable to the measurement errors. To the best of our knowledge, the effect of different crystal phases on interface properties and the Schottky barrier height has not been studied so far. However, according to the present understanding of the Schottky barrier height dependence on material properties [3] , the crystal phase per se does not affect the Schottky barrier height. Instead, the presence of different defects and the specific interface atomic structure determines the barrier height. In our case, the interface between the catalytic particle and semiconductor NW is terminated by As atoms for both (111)B Zinc blende phase and (000-1) Wurtzite phase interfaces, and thus we do not expect any substantial influence of the crystal phase on the Schottky barrier height observed. The epitaxial nature of the Au-catalyst/GaAs-NW interface and its small area are likely responsible for the reduced pinning as chemical bonds form naturally in this epitaxial abrupt junction during the NW growth, which reduces the density of surface states. The small junction area likely also facilitates a relaxation of interfacial defects due to the close proximity of the NW surface [43] . The specific electrostatics for nanoscale contacts is also known to provide weaker impact of metal-induced surface states on the Fermi-level pinning [8] . The reported electric dipole layer contribution to the Schottky barrier height has implications beyond the NW systems studied here. It can also account for the difference in barrier height observed for bulk Schottky contacts formed at semiconductor interfaces with different crystallographic planes. For example, it has been observed for n -type Au/GaAs Schottky contacts that the Schottky barrier is 0.06 eV higher for contacts interfacing with (111)A planes compared with those interfacing with (111)B planes [44] . The observed difference in barrier height is likely to be caused by the electric dipole layers at the contact interface as it corresponds to a realistic density of surface states [40] of 10 18 –10 19 m −2 >>10 17 m −2 . The proposed Schottky barrier-lowering mechanism may also be relevant for contacts formed at abrupt interfaces with thin films with a reduced density of interfacial pinning states, for example, (111)B GaAs grown at low temperature [37] . To the best of our knowledge, this electric dipole layer effect has not been considered before when describing reduced Schottky barrier heights experimentally observed, although similar effects were previously theoretically predicted [3] , [45] . Thus, this finding may be of fundamental importance and can potentially enable Schottky barrier height management by controlling the density of pinning states and by designing the surface dipole layer by choosing appropriate crystal orientation and introducing interfacial atoms with appropriate electronegativity. This is important for different applications where optimization of charge transfer processes at semiconductor surfaces is required, for example, in heterogenous photocatalysis and photochemistry [46] . In particular, this finding can be important for realization of low-ohmic abrupt electrical contacts without the need for contact doping or annealing. This would be a major advantage since doping variability is the key challenge for downscaling of electronic devices. Photocurrent studies In addition to our investigation of ultra-low Schottky barriers formed at Au-catalyst/NW interfaces, the progress in realizing EBL-defined selective contacts to the Au-catalysts opens up the possibility to design and perform new studies combining multiple characterization techniques to probe electron transport at the catalyst/NW epitaxial interface in great detail. In contrast to STM contacting techniques, our approach allows for temperature-dependent and light-assisted I–V measurements, which are typically difficult to perform in STM-based approaches. To demonstrate this versatility, we performed photocurrent measurements on the catalyst/NW epitaxial contacts, which reveal a clear photovoltaic effect and a linear dependence of the short-circuit current on the excitation light power, which is desirable for photodetection applications ( Supplementary Fig. 2 ). The measurements demonstrate that the selective contacts defined with EBL provide the ability to combine multiple characterization techniques for studying the same catalyst/NW epitaxial interface. This is a crucial advantage as quantifying and controlling material properties, such as carrier concentration and mobility by, for example, spatially resolved Hall measurements or electron beam-induced cathodoluminescence measurements on single NWs [47] , are essential for providing more insight into electron transport at nanoscale interfaces and engineering nanoscale electrical contacts with desirable electrical properties. Series A NW growth Series A heterostructure NWs were grown by a custom-built CBE system from Au aerosol seed particles with 70 nm diameter produced by an aerosol method [48] . The particles were deposited on an InAs (111)B substrate with a density of ~0.5 particles per μm 2 . Before the growth, the samples were annealed at 520 °C for 20 min in a tertiarybutylarsine (TBAs) atmosphere in the CBE reactor. The NW growth was carried out at 420 °C using trimethylindium (TMIn), triethylgallium (TEGa) and TBAs as precursors. The source pressures in the lines before the inlet valves during the growth were p As =150 Pa for TBAs, p In =20 Pa for TMIn and p Ga =20 Pa for TEGa. The NWs were grown about 4 μm long, with a resulting diameter of about 90 nm. After growth, precautions were made not to expose the NWs to air for extended periods of time before electrical characterization. Series B NW growth Series B NWs were grown by MOVPE (AIX200/4, Aixtron AG) from Au aerosol seed particles with 80 nm diameter produced by the aerosol method. The particles were deposited on a GaAs (111)B n -type substrate (Si doped, ~10 18 cm −3 doping level) with a density of approximately five particles per μm 2 . Before the growth, the samples were exposed to TMIn for 2 min at 350 °C to enrich the seed particles with In to a level comparable to that of the series A NWs. Subsequently, the samples were annealed at 600 °C for 9 min in hydrogen (H 2 ) and arsine (AsH 3 ) atmosphere in the MOVPE reactor. The NW growth at 450 °C with trimethylgallium (TMGa) and AsH 3 precursors (molar fractions 10 −5 and 10 −4 , respectively) in a H 2 carrier gas flow of 6 × 10 −3 m 3 min −1 resulted in vertical GaAs NWs with a length of up to 500 nm and a diameter of 95 nm. The growth was conducted under low pressure (10 kPa). NW samples with three different doping profiles were grown: fully n -type (Sn doping with an estimated concentration of 10 18 cm −3 was introduced during the whole 2 min NW growth), half-way-doped n -type (Sn doping with an estimated concentration of 10 18 cm −3 was introduced during the first 2 min of the NW growth, followed by a 2 min growth of a nominally undoped NW segment) and nominally undoped. Triethyltin (TESn) was used for the NW doping. After growth, precautions were made not to expose the NWs to air for extended periods of time before electrical characterization. NW inspection with TEM A 300-kV TEM (JEOL JEM-3000F) equipped with a field emission gun was used to characterize the A series NWs with a resolution of 0.165 nm. To prepare the samples for TEM analysis, a Cu grid was rubbed against the substrate surface, which broke off the NWs close to their base. Formation of electrical contacts to series A NWs After growth, NWs from the A series were mechanically transferred onto silicon substrates capped with a thermally grown 100 nm thick silicon dioxide top layer. The substrates had a set of macroscopic metal pads for connection to the external circuitry. The substrates also had predefined reference markers for accurate location of the NWs and alignment crosses for subsequent EBL alignment. The reference markers and the alignment crosses were made in an EBL process (Raith 150 EBL system, Raith GmbH) by thermal evaporation of 10 nm Ti and 50 nm Au with a subsequent lift-off process. EBL was used to define selective electrical contacts to the Au-catalyst nanoparticle and to the InAs segment of single NWs. To form selective electrical contacts to Au-catalyst nanoparticles, it was crucial to perform a high-precision alignment of the metal electrodes formed by EBL with respect to the mechanically deposited NWs. For this, the position of individual NWs, relative to the reference markers, was determined by taking images with the SEM of the EBL system. The images were recorded at 20 kV accelerating voltage with a maximum radiation dose limited to ~700 μC cm −2 , as it was observed that higher doses could damage the NWs. Before recording each image, a field alignment was done using the predefined alignment markers. The specific design ( Supplementary Fig. 3 ) of the reference markers and the alignment crosses, including features with dimensions down to 40 nm, was important for the high-precision alignment process. The sample was coated with a standard e-beam-sensitive resist polymethylmethacrylate (PMMA) after localizing NWs of interest. A 150 nm thick single layer of PMMA (molecular weight 950,000 Da) was deposited by spinning at 5,000 r.p.m. for 30 s with a subsequent baking at 180 °C for 1 h in an oven. The EBL exposure was done at 20 kV accelerating voltage with a 700 μC cm −2 radiation dose. The high-precision NW alignment carried out before the electron beam exposure allowed a control of the electric contact position to within 10–20 nm, see inset in Fig. 2 . The yield of the selective contacts was found to be up to 80% and was mostly limited by NW displacement during the e-beam resist spinning. A second EBL step was subsequently carried out to establish the ohmic contact to the InAs segment of the NW and included InAs surface sulphur passivation [17] . The contacts to the Au particle and InAs segment were both fabricated by thermal evaporation of 250 Å Ni and 900 Å Au with a subsequent lift-off process. Barrier height analysis for series A NWs The ideal I-V relation for a metal–semiconductor contact under TE conditions is given by [1] where J is the current density per unit area, A * is the Richardson constant, q ϕ E is the effective potential barrier height and V app is the bias applied, positive for forward bias, that is, positive potential applied to the metal side. For V app <− 3 kT/q and a bias-dependent effective barrier height q ϕ E ( V app ), equation (3) reduces to which can be rewritten in the form for barrier height analysis from Arrhenius plots, I is the current through the device and A is the effective contact area. Here it is assumed that the quasi-Fermi level for electrons remains horizontal throughout the depletion region. This assumption is valid if the electron mean free path exceeds the distance within which the barrier falls by kT/q from its maximum value [1] . This is likely the case for our study as we have high-mobility materials and from previous studies the mean free path is known to exceed 50 nm for similar semiconductor NW systems [49] . In addition, the barrier height is assumed to be temperature-independent [19] . This is likely the case for our study as we obtain straight lines in the Arrhenius plots, see Fig. 3b . Band diagram reconstruction for series A NWs The band diagram reconstruction was done by solving the one-dimensional Poisson equation at zero bias and 300 K (ref. 20 ). We used bulk material parameters, since the Fermi wavelength of electrons in the NWs is much smaller than the NW diameter [49] . In accordance with TEM studies, the GaAs segment length was taken to be 25 nm and the InGaAs transition region to be 80 nm. InAs was considered to be n -type with a doping concentration of 10 17 cm −3 , and GaAs was considered to be p -type with the same doping concentration. The doping concentration was interpolated for the graded InGaAs segment. Indeed, it was previously demonstrated that epitaxial InAs NWs are unintentionally degenerately n -type doped (10 17 cm −3 ) [29] , whereas GaAs NWs become p -type. Residual carbon was suggested to be the source of doping in both InAs and GaAs NWs, in agreement with the amphoteric behaviour of carbon [30] . Barrier height analysis for series B NWs Series B NWs with different doping profiles (fully n -type, half-way-doped n -type and nominally undoped) were characterized with I-V measurements using STM [33] . Several NWs of the same type were characterized in this way. For STM characterization, the exact position of as-grown GaAs NWs standing vertically on the substrate was first determined with the STM [50] . Subsequently, the STM tip was gently pressed directly into the catalytic Au particle of an individual GaAs NW, with a precaution not to damage the NW [51] . By this procedure an ohmic point contact between the metallic STM tip (etched tungsten wire sputtered in vacuum) and the catalytic particle was established [51] . The GaAs substrate was used as the other contact for the I–V measurements. The STM system allowed electrical characterization only at room temperature (300 K) in darkness. The accuracy of the Schottky barrier height extraction with this method is limited by the uncertainty of Richardson’s constant [19] . For our analysis, A *=7±3 A cm −2 K −2 was extracted from Arrhenius plots of the A series samples for V app >0. This value is comparable to the values theoretically predicted [52] and experimentally observed for GaAs [53] , [54] . We obtained q ϕ S =0.32±0.04 eV for nominally undoped NWs from series B . For fully n -type NWs the electrical current was a few orders of magnitude higher than that for half-way-doped n -type NWs and there was almost no rectification indicating that the interface between free-standing GaAs NWs and GaAs substrate did not affect our Schottky barrier height measurements for half-way-doped n -type NWs. Furthermore, the same Schottky barrier height was obtained for half-way-doped n -type and nominally undoped NWs indicating that the interface between free-standing GaAs NWs and GaAs substrate also did not affect our Schottky barrier height measurements for nominally undoped NWs. Using the same analysis method of extracting the barrier height at 300 K on series A NWs gives a barrier height of 0.56±0.03 eV, which is consistent with the zero bias barrier in Fig. 3c . Electric dipole layer influence on the Schottky barrier The electric dipole layer is formed because of the termination of the GaAs NW by As atoms at the contact interface with the Au catalyst. In the following, we estimate the potential energy difference caused by the electric dipole layer, qd ϕ . According to the Pauling scale, the electronegativity of Ga and As is 1.77 and 2.25, respectively [55] , and the ionicity of the Ga–As chemical bond in GaAs amounts to ω =0.31 (ref. 56 ). The electronegativity difference leads to an electric dipole layer formation at the Au-catalyst/GaAs-NW interface with a step in the electric potential. Let us consider the electric dipole layer as a parallel plate capacitor with a corresponding capacitance , where ∈ 0 =8.85 × 10 −12 F m −1 is the dielectric constant, A is the effective contact area between the catalytic particle and the NW and l is the thickness of the electric dipole layer. Using the definition of electric capacitance C=Q/dϕ , where Q is the charge at a potential difference dϕ , we can rewrite the capacitor equation as The electric dipole layer can be characterized by its dipole moment μ = q e l , where q e is the effective electric charge and | l |= l can be calculated from the crystal structure of GaAs as =2.45 Å, where a =5.65 Å is the lattice constant of GaAs [19] . Taking into account the chemical bond ionicity, equation (6) can be written in the following form: where N s =8.85 × 10 18 m −2 is the atomic surface density as calculated from the crystal structure of GaAs and q e =0.2· q =3.2 × 10 −20 C is the effective electric charge for one Ga-As ionic bond [57] . Equation (7) yields the potential difference dϕ =2.43 V, which corresponds to a potential energy difference qd ϕ =2.43 eV. The ideal Schottky model ( Fig. 5a ) predicts a Schottky barrier for the In-alloyed Au-catalyst/GaAs-NW interface of q ϕ S(AuIn) = q ϕ AuIn – q χ GaAs =0.89 eV ( q ϕ AuIn =4.96 eV is the work function for an AuIn alloy with an In content of 30 at.% (ref. 39 ), q χ GaAs =4.07 eV (ref. 38 ) is the affinity for GaAs). The electric field associated with the formed electric dipole layer leads to a step in the potential energy at the interface (As atoms in contact with Au-catalyst have higher electronegativity than Ga atoms). In the ideal Schottky model, this step shifts the conduction band edge of GaAs below the Fermi level in the Au-catalyst particle ( Fig. 5b ) by an amount q Δ=0.5· qd ϕ –q ϕ S(AuIn) =0.33 eV. From our experiments we extract a Schottky barrier height between the Au-catalyst and GaAs NW of q ϕ S =0.35 eV. We now assume that pinning states at the interface account for the potential energy qd ϕ States =q ϕ S + q Δ=0.68 eV. From this assumption, the density of pinning states can readily be estimated if we again consider an electric dipole layer, now formed by the surface states and the charges induced by them in the metal particle [5] . If we substitute Q/A=n·q in equation (6), where n is the density of surface states, then n can be assessed as: Equation (8) yields a surface density of states ~10 17 m −2 at the Au-catalyst/GaAs interface. How to cite this article: Suyatin, D. B. et al. Strong Schottky barrier reduction at Au-catalyst/GaAs-nanowire interfaces by electric dipole formation and Fermi-level unpinning. Nat. Commun. 5:3221 doi: 10.1038/ncomms4221 (2014).